BMP signalling regulates the pre-implantation development of extra-embryonic cell lineages in the mouse embryo Pre-implantation development requires the specification and organization of embryonic and extra-embryonic lineages. The separation of these lineages takes place when asymmetric divisions generate inside and outside cells that differ in polarity, position and fate. Here we assess the global transcriptional identities of these precursor cells to gain insight into the molecular mechanisms regulating lineage segregation. Unexpectedly, this reveals that complementary components of the bone morphogenetic protein (BMP) signalling pathway are already differentially expressed after the first wave of asymmetric divisions. We investigate the role of BMP signalling by expressing dominant negative forms of Smad4 and Bmpr2, by downregulating the pathway using RNA interference against BMP ligands and by applying three different BMP inhibitors at distinct stages. This reveals that BMP signalling regulates the correct development of both extra-embryonic lineages, primitive endoderm and trophectoderm, but not the embryonic lineage, before implantation. Together, these findings indicate multiple roles of BMP signalling in the early mouse embryo. Pre-implantation development results in the formation of a blastocyst comprising three distinct cell lineages: the trophectoderm (TE), primitive endoderm (PE) and epiblast (EPI). The specification of these lineages is initiated when a subset of cells are directed to the inside of the embryo during two major waves of asymmetric divisions at the 8- to 16-cell and 16- to 32-cell transitions [1] . Cells on the outside of the embryo are destined to differentiate into extra-embryonic TE, whereas inside cells form the pluripotent inner cell mass (ICM). Cells of the ICM will become either the pluripotent EPI that will give rise to the fetus or the PE that contributes predominantly to extra-embryonic tissues. Understanding of the molecular events underlying pre-implantation development has been significantly improved by several recent single-cell microarray and RNA-sequencing studies [2] , [3] , [4] . However, the transcriptional identities of the first progenitors of the TE (outside cells) and the ICM (inside cells) currently remain unknown. Early asymmetries in ligand/receptor expression could indicate involvement in later cell fate decisions, as has been shown recently for differential expression of Fgfr2 and Fgf4 (refs 5 , 6 ), but the involvement of other key signalling pathways in lineage segregation is unclear [7] . For example, the BMP signalling pathway is critical for development and patterning in many developmental systems [8] , [9] . In the mouse, BMP signalling is known to regulate several aspects of early post-implantation development, including germ cell differentiation and anterior–posterior patterning [10] , [11] , [12] , [13] , [14] , [15] , and to drive TE differentiation in vitro [16] . However, studies showing that mice lacking core BMP signalling pathway components do not arrest embryogenesis until after implantation suggested that BMP signalling might be dispensable for pre-implantation development [10] , [11] , [17] , [18] . Here, with an aim to investigate the mechanisms involved in the first steps leading to lineage segregation in the mouse embryo, we used deep mRNA sequencing to identify the transcripts expressed in inside and outside cells as they first become set apart at the 16-cell stage. Analysis of this data set pointed to an unexpected role of BMP signalling in pre-implantation development. To test this hypothesis, we inhibited BMP signalling in the embryo using six distinct and independent approaches. Our results indicate that BMP signalling is important much earlier in development than previously expected and that it is key for the development of both pre-implantation extra-embryonic lineages. Expression of BMP pathway components at the 16-cell stage To investigate the first steps leading to lineage segregation in the mouse embryo, we first wished to determine global differences in gene expression between inside and outside cells after the first wave of asymmetric cell divisions ( Fig. 1a ). To isolate these cells, we incubated early 16-cell stage embryos in a suspension of 0.2 μm fluorescent beads ( Supplementary Fig. 1 ) and then used gentle pipetting to separate inside (non-fluorescent) and outside (fluorescent) cells ( Fig. 1b ). We combined 30–40 cells of the same identity and performed mRNA deep sequencing on the SOLiD platform, using the protocol developed for low cell number samples [19] . Colour-space reads obtained were mapped to the mouse genome and all reads that mapped to particular genes in either cell type were summed. We applied the GFOLD (generalized fold change) algorithm [20] to obtain biologically meaningful rankings of differentially expressed genes ( Supplementary Fig. 2 and Supplementary Data 1 and 2 ). We found that more than 11,000 transcripts from the mouse RefSeq database were expressed in either cell type. 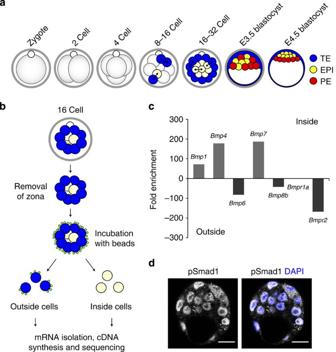Figure 1: Transcriptome analysis of inside and outside cells at the 16-cell stage. (a) Schematic representation of pre-implantation development. Briefly, two waves of asymmetric divisions at the 8- to 16- and 16- to 32-cell transitions set apart the outside progenitors of the TE (blue) and the inside progenitors of the ICM (pale yellow). Cells of the ICM will further segregate into the EPI and PE in the late blastocyst. (b) Isolation and deep sequencing of outside and inside cells from the 16-cell embryo. (c) BMP ligands and receptors differentially expressed at the 16-cell stage. (d) pSmad1 expression in the early blastocyst. Scale bars, 40 μm. Transcripts from about 10% of these genes were enriched more than 5-fold (GFOLD≤0.01) in one cell type ( Supplementary Table 1 ). To verify our findings, we assessed the expression levels of Id2 and Sox2 , genes reported to be early markers of outside and inside cells, respectively [2] , and found that they were enriched in the expected cell type, with Id2 enriched 4-fold more in outside cells (outside:inside=613:149) and Sox2 enriched 39-fold more in inside cells (9:355). We also quantified relative expression levels between inside and outside cells for 46 genes by quantitative reverse transcription–PCR (qRT–PCR; Supplementary Fig. 3 ), which further validated the differential expression. We wished to determine whether other genes involved in maintaining pluripotency in the ICM, or driving differentiation in the TE and PE, in addition to Sox2 and Id2 , are already differentially expressed after the first wave of asymmetric divisions. We found that transcripts for Cdx2 (748:413) [21] , [22] and Gata3 (5,746:1,086) [23] are enriched in outside cells, whereas Fgf4 (3:322) [24] , [25] is expressed 100-fold more in inside cells. Figure 1: Transcriptome analysis of inside and outside cells at the 16-cell stage. ( a ) Schematic representation of pre-implantation development. Briefly, two waves of asymmetric divisions at the 8- to 16- and 16- to 32-cell transitions set apart the outside progenitors of the TE (blue) and the inside progenitors of the ICM (pale yellow). Cells of the ICM will further segregate into the EPI and PE in the late blastocyst. ( b ) Isolation and deep sequencing of outside and inside cells from the 16-cell embryo. ( c ) BMP ligands and receptors differentially expressed at the 16-cell stage. ( d ) pSmad1 expression in the early blastocyst. Scale bars, 40 μm. Full size image It has recently been established that differential expression of Fgf4 and Fgfr2 at the 16-cell stage is important for regulating segregation of the EPI and PE lineages within the ICM [5] , [6] . This prompted us to determine whether ligands or receptors of any other signalling pathways might also show differential expression at the 16-cell stage and led us to focus on the BMP pathway ( Fig. 1c ). We found that while inside cells express Bmp4 (0:89) and Bmp7 (0:94), outside cells express Bmp6 (41:0) and Bmp8b (393:9). Bmpr1a , which encodes the receptor that binds Bmp4 and 7, is expressed in both inside and outside cells at similar levels (566:546). However, mRNA for Bmpr2 , necessary for signal transduction, is expressed exclusively in outside cells (84:0), suggesting that the outside cells are the predominant recipients of the signal. These early differential expression patterns correlate with the expression of Bmpr2 and Bmp4/Bmp7 at later developmental stages in the same reciprocal outside/inside pattern in TE and ICM cells of the blastocyst [3] . BMP signalling can occur via both Smad-dependent and -independent pathways [26] and we detected mRNAs for components of both downstream signalling routes in outside and inside cells, including Smad4 (1172:936), Smurf1 (809:826) and Tak1 (556:636). To confirm that the BMP signalling pathway is active in the pre-implantation embryo, we determined the localization of pSmad1 at the early blastocyst stage ( Fig. 1d ). We found that nuclear pSmad1 was present at this stage, in agreement with previous work showing nuclear pSmad1 in the TE and PE of the late blastocyst [27] . The differential expression of BMP pathway ligands and receptors at the 16-cell stage prompted us to investigate whether BMP signalling might play a role in development before embryo implantation. Inhibition of Smad4 and Bmpr2 in the pre-implantation embryo To determine whether BMP signalling is involved in pre-implantation development, we first used dominant negative forms of Smad4 (dnSmad4) and Bmpr2 (dnBmpr2) to inhibit the BMP/Smad4 pathway in vivo . We injected one blastomere of late two-cell stage embryos with mRNA for either dnSmad4 or dnBmpr2 , along with mRNA for membrane-bound red fluorescent protein (RFP) ( Gap43-RFP ) as a lineage marker of the injected clone of cells. The half of the embryo developing from the non-injected blastomere provided an internal control. An additional group of control embryos were injected with Gap43-RFP alone. The embryos were then cultured for 3 days to the late blastocyst stage (E4.5), and the contribution of Gap43-RFP-expressing cells to each lineage assessed by immunofluorescence for lineage markers of the TE (Cdx2) and PE (Sox17; Fig. 2a ). As the red channel was required for visualizing the Gap43-RFP expression, EPI cells were counted as those that were negative for both Cdx2 and Sox17. We found that expression of both dominant negatives resulted in significantly fewer cells in the injected half of the embryo, by 22% for dnSmad4 ( P <0.001, Student’s t -test) and by 23% for dnBmpr1 ( P <0.001, Student’s t -test), compared with controls ( Fig. 2b,c ). This reduction in total cell number could be entirely attributed to a reduced number of TE and PE cells, with the number of EPI cells either increased for dnSmad4 (by 47%, P <0.05, Student’s t -test) or not significantly affected for dnBmpr2. Expression of dnSmad4 resulted in a 28% decrease in TE cells ( P <0.001, Student’s t -test) and a 44% decrease in PE cells ( P <0.001, Student’s t -test), whereas expression of dnBmpr2 reduced TE cells by 29% ( P <0.001, Student’s t -test) and PE cells by 29% ( P <0.05, Student’s t -test). Although control injected ICM cells contributed roughly equally to the EPI and PE (56% PE), ICM cells with dnSmad4 (33% PE, P <0.001, Student’s t -test) or dnBmpr2 (40% PE, P <0.01, Student’s t -test) showed reduced contribution to the PE lineage ( Fig. 2d ). These results suggest an important involvement of BMP signalling in pre-implantation development and specifically in the development of the extra-embryonic lineages: the TE and PE. 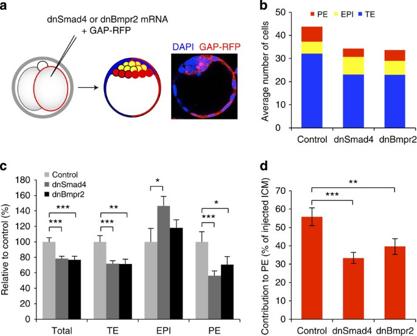Figure 2: Expression of dominant negative forms of Smad4 and Bmpr2 affects TE and PE development. (a) One blastomere of two-cell embryos was injected withdnSmad4(n=21),dnBmpr2(n=22) orGap43-RFPonly (controlsn=20) and cultured to E4.5. (b) Total cell numbers for each lineage in the injected (Gap43-RFP-positive) half of the embryo. (c) Total cell numbers and lineage contributions relative to control. (d) Contribution of injected ICM cells to PE. *P<0.05, **P<0.01, ***P<0.001 (Student’st-test). Error bars represent s.e.m. Figure 2: Expression of dominant negative forms of Smad4 and Bmpr2 affects TE and PE development. ( a ) One blastomere of two-cell embryos was injected with dnSmad4 ( n =21), dnBmpr2 ( n =22) or Gap43-RFP only (controls n =20) and cultured to E4.5. ( b ) Total cell numbers for each lineage in the injected (Gap43-RFP-positive) half of the embryo. ( c ) Total cell numbers and lineage contributions relative to control. ( d ) Contribution of injected ICM cells to PE. * P <0.05, ** P <0.01, *** P <0.001 (Student’s t -test). Error bars represent s.e.m. Full size image BMP inhibition impairs development of the TE and PE lineages Blocking the activity of Smad4 and Bmpr2 suggested that BMP signalling might play a role in the development of the extra-embryonic lineages before implantation. We sought to confirm this finding by alternative methods of BMP inhibition. To do this, we used three specific inhibitors to block either the Smad-dependent or -independent BMP pathways in vivo : Noggin, a BMP ligand antagonist [28] ; Dorsomorphin, an inhibitor of Bmpr1 that leads to inhibition of Smad1 phosphorylation [29] and the Tak1 kinase inhibitor (5Z)-7-Oxozeaenol that inhibits the Smad-independent response to BMPs [30] . Embryos were cultured in the presence of the inhibitors from the eight-cell stage (E2.5) to the late blastocyst stage (E4.5) and assessed for the expression of markers of the TE (Cdx2), EPI (Nanog) and PE (Sox17; Fig. 3a ). Each inhibitor was used at two different concentrations to determine if any effects on development were dose dependent. We found that all three inhibitors caused a significant reduction in the number of Sox17-positive PE cells compared with control embryos, in a dose-dependent manner (Noggin (150 ng ml −1 ), 20% less PE, P <0.05, Student’s t -test; Noggin (300 ng ml −1 ), 47% less PE, P <0.001, Student’s t -test; (5Z)-7-Oxozeaenol (250 nM), 20% less PE, P <0.05, Student’s t -test; (5Z)-7-Oxozeaenol (500 nM), 65% less PE, P <0.001, Student’s t -test; Dorsomorphin (0.5 μM), 67% less PE, P <0.001, Student’s t -test; Dorsomorphin (1.0 μM), 91% less PE, P <0.001, Student’s t -test; Fig. 3b–e ). A decrease in the total number of cells in the embryos compared with controls (98.5 cells) was observed for the higher concentrations of Noggin (by 11%, 87.3 cells, P <0.05, Student’s t -test) and Dorsomorphin (by 17%, 81.7 cells, P <0.001, Student’s t -test), however, (5Z)-7-Oxozeaenol treatment did not significantly affect total cell number. All higher concentration treatments resulted in a decrease in TE cells, by 11% for Noggin ( P =0.07, Student’s t -test), by 13% for (5Z)-7-Oxozeaenol ( P <0.01, Student’s t -test) and by 9% for Dorsomorphin ( P <0.05, Student’s t -test). Both Noggin and Dorsomorphin had an effect only on the development of the TE and PE lineages, but not on the EPI lineage. The only inhibitor to have a significant effect on the number of Nanog-positive EPI cells was (5Z)-7-Oxozeaenol, which caused a significant increase in Nanog-positive cells in a dose-dependent manner, by 24% at 250 nM ( P <0.05, Student’s t -test) and by 81% at 500 nM ( P <0.001, Student’s t -test). 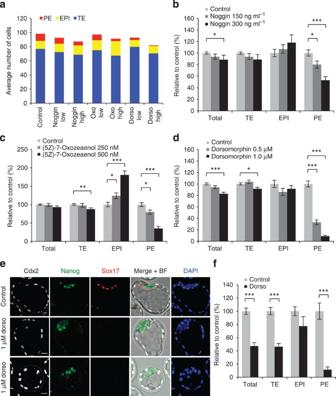Figure 3: BMP inhibitor treatments reduce the number of extra-embryonic cells at E4.5. (a–e) Embryos were incubated in the presence of BMP inhibitors for 48 h from E2.5 to E4.5. Controls,n=37; 150 ng ml−1of Noggin,n=23; 300 ng ml−1of Noggin,n=12; 250 nM (5Z)-7-Oxozeaenol,n=27; 500 nM (5Z)-7-Oxozeaenol,n=16; 0.5 μM Dorsomorphin,n=25; 1.0 μM Dorsomorphin,n=47. (a) Total cell numbers for each lineage at E4.5. (b–d) Total cell numbers and lineage contributions relative to control embryos. (e) Immunofluorescence for markers of the TE (Cdx2), EPI (Nanog) and PE (Sox17) in embryos treated with 1.0 μM Dorsomorphin. Scale bars, 20 μm. (f) Relative number of cells in each lineage compared with controls (n=10) in embryos treated with 1.0 μM Dorsomorphin (n=10) for 72 h from E1.5 to E4.5. *P<0.05, **P<0.01, ***P<0.001 (Student’st-test). Error bars represent s.e.m. Figure 3: BMP inhibitor treatments reduce the number of extra-embryonic cells at E4.5. ( a – e ) Embryos were incubated in the presence of BMP inhibitors for 48 h from E2.5 to E4.5. Controls, n =37; 150 ng ml −1 of Noggin, n =23; 300 ng ml −1 of Noggin, n =12; 250 nM (5Z)-7-Oxozeaenol, n =27; 500 nM (5Z)-7-Oxozeaenol, n =16; 0.5 μM Dorsomorphin, n =25; 1.0 μM Dorsomorphin, n =47. ( a ) Total cell numbers for each lineage at E4.5. ( b – d ) Total cell numbers and lineage contributions relative to control embryos. ( e ) Immunofluorescence for markers of the TE (Cdx2), EPI (Nanog) and PE (Sox17) in embryos treated with 1.0 μM Dorsomorphin. Scale bars, 20 μm. ( f ) Relative number of cells in each lineage compared with controls ( n =10) in embryos treated with 1.0 μM Dorsomorphin ( n =10) for 72 h from E1.5 to E4.5. * P <0.05, ** P <0.01, *** P <0.001 (Student’s t -test). Error bars represent s.e.m. Full size image Inhibition of BMP signalling by the use of specific inhibitors again indicated a role of the BMP pathway in the development of both extra-embryonic cell lineages; however, we noticed that targeting the activity of Smad4 and Bmpr2 had a greater effect on the TE lineage than the inhibitors. To determine whether this greater effect on the TE was due to the different start points of each experiment, from late two-cell stage in the case of dnSmad4 and dnBmpr2 and from the eight-cell stage in the inhibitor treatments, we next cultured embryos in 1.0 μM Dorsomorphin from the late two-cell stage for 72 h and analysed lineage-specific gene expression at E4.5, compared with controls ( Fig. 3f ). This longer Dorsomorphin treatment had a much more severe effect on the number of total (reduced by 53%, P <0.001, Student’s t -test) and TE (reduced by 54%, P <0.001, Student’s t -test) cells than the previous 48 h treatment. The number of EPI cells was not significantly different to controls and the PE was reduced by 89% ( P <0.001, Student’s t -test), consistent with previous experiments. Together, these results demonstrate that inhibition of BMP signalling causes a defect specifically in the development of the extra-embryonic lineages of the blastocyst. Cell death in BMP inhibitor-treated embryos To gain insight into the mechanism by which inhibition of BMP signalling prevents normal development of extra-embryonic lineages, we assessed whether programmed cell death might play a role. Embryos were treated with 300 ng ml −1 of Noggin, 500 nM (5Z)-7-Oxozeaenol or 1.0 μM Dorsomorphin from E2.5 to E4.5 and examined for the expression of cleaved caspase 3 ( Fig. 4a,b ). We found that the average percentage of cells expressing cleaved caspase 3 in each embryo was significantly increased by 4.6-fold for Noggin ( P <0.05, Student’s t -test) and by 10.6-fold for Dorsomorphin ( P <0.001, Student’s t -test), compared with control embryos. Embryos treated with (5Z)-7-Oxozeaenol showed a slight, but not quite significant ( P =0.05, Student’s t -test) increase in the percentage of cells expressing cleaved caspase 3, suggesting that in these embryos another mechanism may be responsible for the decrease in extra-embryonic cells. The increased presence of apoptotic cells in embryos treated with Noggin or Dorsomorphin could indicate a pro-survival role of BMP signalling during pre-implantation development. To investigate whether BMP signalling inhibited apoptosis, we assessed whether BMP4 treatment could inhibit actinomycin D-induced cell death in pre-implantation embryos [31] . Eight-cell stage embryos were treated with a low concentration of actinomycin D (2 ng ml −1 ) for 6 h, then washed in normal media and cultured for 48 h to E4.5. Throughout the experiment, half of the embryos were cultured in the presence of exogenous BMP4 to determine whether this would affect cell survival ( Fig. 4c ). We found that the addition of BMP4 did not increase the number of cells in actinomycin D-treated embryos, suggesting that BMP signalling does not inhibit apoptosis and that the cell death observed in Dorsomorphin- and Noggin-treated embryos is most likely secondary to a developmental defect. 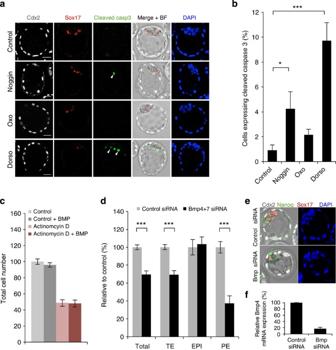Figure 4: Mechanisms of extra-embryonic cell loss in embryos with impaired BMP signalling. (a) Examples of cleaved caspase 3 expression in embryos treated with 300 ng ml−1of Noggin (n=12), 500 nM (5Z)-7-Oxozeaenol (n=15) or 1.0 μM Dorsomorphin (n=15) for 48 h from E2.5 to E4.5 (controls,n=14). White arrows indicate examples of apoptotic cells. (b) Percentage of cells per embryo that express cleaved caspase 3. (c) Total cell number relative to controls (n=12) in E4.5 stage embryos treated with BMP4 (n=12), actinomycin D (n=17) or actinomycin D+BMP4 (n=17). (d) Number of cells in each lineage at E4.5 in embryos injected withBmp4+7siRNA (n=13), relative to controls (n=12). (e) Examples of E4.5 embryos, 72 h after microinjection with siRNA. (f) Confirmation of Bmp4 knockdown by qRT–PCR 48 h after siRNA injection.BmpsiRNA,n=50; controls,n=50 (three experiments). Scale bars, 30 μm. *P<0.05, ***P<0.001 (Student’st-test). Error bars represent s.e.m. Figure 4: Mechanisms of extra-embryonic cell loss in embryos with impaired BMP signalling. ( a ) Examples of cleaved caspase 3 expression in embryos treated with 300 ng ml −1 of Noggin ( n =12), 500 nM (5Z)-7-Oxozeaenol ( n =15) or 1.0 μM Dorsomorphin ( n =15) for 48 h from E2.5 to E4.5 (controls, n =14). White arrows indicate examples of apoptotic cells. ( b ) Percentage of cells per embryo that express cleaved caspase 3. ( c ) Total cell number relative to controls ( n =12) in E4.5 stage embryos treated with BMP4 ( n =12), actinomycin D ( n =17) or actinomycin D+BMP4 ( n =17). ( d ) Number of cells in each lineage at E4.5 in embryos injected with Bmp4+7 siRNA ( n =13), relative to controls ( n =12). ( e ) Examples of E4.5 embryos, 72 h after microinjection with siRNA. ( f ) Confirmation of Bmp4 knockdown by qRT–PCR 48 h after siRNA injection. Bmp siRNA, n =50; controls, n =50 (three experiments). Scale bars, 30 μm. * P <0.05, *** P <0.001 (Student’s t -test). Error bars represent s.e.m. Full size image Source of BMP signals in the pre-implantation embryo Our finding that both inside and outside cells express Bmp ligands led us to investigate which cells are the source of the BMP signals important for the development of the TE and PE. To do this, we used short interfering RNA (siRNA) to knockdown the expression of Bmp4 and Bmp7 as these two ligands are exclusively produced by inside cells at the 16-cell stage and by the ICM in the blastocyst [2] , [3] , [32] . Both blastomeres of two-cell stage embryos were injected with Bmp4+7 siRNA or control siRNA and the embryos cultured for 72 h to the late blastocyst stage ( Fig. 4d,e ). We found that the Bmp4+7 siRNA-injected embryos had 30% less total cells than control siRNA-injected embryos ( P <0.001, Student’s t -test) and that this was due to a decrease in the number of TE cells (by 31%, P <0.001, Student’s t -test) and PE cells (by 63%, P <0.001, Student’s t -test). The number of EPI cells did not differ between the two groups of embryos. To confirm the knockdown of Bmp4 and Bmp7, both blastomeres of two-cell stage embryos were injected with Bmp4+7 siRNA or control siRNA and the levels of Bmp4 and 7 mRNA analysed 48 h later, at E3.5 ( Fig. 4f ). Transcripts for Bmp4 were depleted by 83% compared with controls, however, Bmp7 could not be detected, most likely due to its low expression at this stage [33] . These results indicate that BMP signals produced by the pluripotent inside cells are important for the development of the extra-embryonic TE and PE lineages. Mechanism of PE cell loss in Dorsomorphin-treated embryos Dorsomorphin treatment had the strongest effect on Sox17-positive PE cell number; therefore, we checked the expression of other PE-specific genes in embryos treated with 1.0 μM Dorsomorphin from E2.5 to E4.5 ( Supplementary Fig. 4 ). We found that the expression of two other PE markers, Gata6 and Gata4, was markedly reduced compared with controls, confirming compromised development of PE. To further investigate this, we analysed the expression of early markers of PE and EPI (Gata6 and Nanog, respectively) in E4.5 blastocysts treated with 1.0 μM Dorsomorphin from E2.5, compared with controls ( Fig. 5a ). We found that the number of Gata6-positive cells was reduced by 78% ( P <0.001, Student’s t -test) and the overall number of ICM cells was reduced by 37% ( P <0.001, Student’s t -test), however, the number of cells expressing Nanog was not significantly affected ( Fig. 5b ). This suggests that PE precursor cells are either eliminated by cell death or never specified. Quantification of the cleaved caspase 3 staining indicates that there is a dramatically increased occurrence of cell death in Dorsomorphin-treated embryos (with almost 10% of cells in the blastocyst expressing cleaved caspase 3; Fig. 4b ) and the presence of dying cells on the surface of the ICM supports the hypothesis that PE cells are actively eliminated ( Fig. 5c ). To determine whether PE precursor cells are specified in the early ICMs of Dorsomorphin-treated embryos, we assessed Gata6 and Nanog expression at E3.5 in embryos treated with 1.0 μM Dorsomorphin from E2.5 ( Fig. 5d ). We found that at this stage around half of ICM cells expressed both Gata6 and Nanog in both controls and Dorsomorphin-treated embryos. There was a reduction in the number of ICM cells expressing only Gata6 in Dorsomorphin-treated embryos (by 43%, 2.4 cells compared with 4.3 cells, P <0.05, Student’s t -test; Fig. 5d ), however, this did not significantly affect the total number of ICM cells (19.9 cells compared with 23.4 cells, P =0.05, Student’s t -test; Fig. 5e ). This reduction of Gata6-positive cells at E3.5 is therefore unlikely to be sufficient to account for the almost complete loss of PE cells at E4.5. 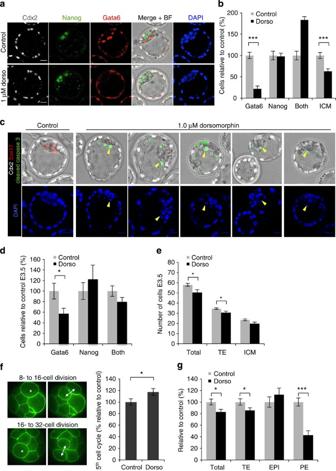Figure 5: Mechanism of PE cell loss in Dorsomorphin-treated embryos. (a–c) Embryos were treated with 1.0 μM Dorsomorphin (n=15) for 48 h from E2.5 to E4.5 (controls,n=15). (a) Expression of Cdx2, Gata6 and Nanog at E4.5. (b) Number of cells relative to controls at E4.5. Both=Cells positive for both Gata6 and Nanog. (c) Examples of dying cells on surface of ICM (identified by cleaved caspase 3 expression and DNA fragments, yellow arrows) at E4.5. (d,e) Embryos were cultured in the presence of 1.0 μM Dorsomorphin (n=16) for 24 h from E2.5 to E3.5 (controls,n=16). (d) Number of cells relative to controls at E3.5. (e) Number of cells in each lineage at E3.5. (f) Time taken for individual cells to complete the fifth cell cycle in embryos cultured with 1.0 μM Dorsomorphin (n=17 cells, 6 embryos) for 48 h from E2.5, relative to controls (n=23 cells, 5 embryos). (g) Number of cells in each lineage relative to controls at E4.5 following treatment with 1.0 μM Dorsomorphin for 24 h from E3.5. Scale bars, 20 μm. *P<0.05, ***P<0.001 (Student’st-test). Error bars represent s.e.m. See alsoSupplementary Fig. 4. Figure 5: Mechanism of PE cell loss in Dorsomorphin-treated embryos. ( a – c ) Embryos were treated with 1.0 μM Dorsomorphin ( n =15) for 48 h from E2.5 to E4.5 (controls, n =15). ( a ) Expression of Cdx2, Gata6 and Nanog at E4.5. ( b ) Number of cells relative to controls at E4.5. Both=Cells positive for both Gata6 and Nanog. ( c ) Examples of dying cells on surface of ICM (identified by cleaved caspase 3 expression and DNA fragments, yellow arrows) at E4.5. ( d , e ) Embryos were cultured in the presence of 1.0 μM Dorsomorphin ( n =16) for 24 h from E2.5 to E3.5 (controls, n =16). ( d ) Number of cells relative to controls at E3.5. ( e ) Number of cells in each lineage at E3.5. ( f ) Time taken for individual cells to complete the fifth cell cycle in embryos cultured with 1.0 μM Dorsomorphin ( n =17 cells, 6 embryos) for 48 h from E2.5, relative to controls ( n =23 cells, 5 embryos). ( g ) Number of cells in each lineage relative to controls at E4.5 following treatment with 1.0 μM Dorsomorphin for 24 h from E3.5. Scale bars, 20 μm. * P <0.05, *** P <0.001 (Student’s t -test). Error bars represent s.e.m. See also Supplementary Fig. 4 . Full size image The number of total (50.4 compared with 58.0, P <0.05, Student’s t -test) and TE (30.6 compared with 34.5, P <0.05, Student’s t -test) cells were both significantly decreased by Dorsomorphin treatment ( Fig. 5e ), indicating that the development of these embryos might be delayed. To determine whether Dorsomorphin treatment indeed causes a developmental delay, we cultured embryos expressing a GFP-tagged membrane protein (GFP-GPI) from E2.5 to E3.5 in 1.0 μM Dorsomorphin and used time-lapse microscopy to film developmental progression. To establish whether Dorsomorphin treatment affects cell cycle time, we measured the time taken for individual cells to undertake the fifth cell cycle (from the 8- to 16-cell division to the 16- to 32-cell division; Fig. 5f ). We found a significant increase in the length of this cell cycle (by 17%, P <0.05, Student’s t -test), compared with control embryos. Dorsomorphin treatment therefore causes a developmental delay that contributes to decreased cell numbers in the extra-embryonic lineages by E4.5. Importantly, our analyses revealed that the embryonic EPI cells are able to escape the effects of this delay as their numbers are not significantly decreased by any of the three inhibitors. Finally, we sought to determine the extent to which the inhibition of BMP signalling between E2.5 and E3.5 contributes to the loss of PE cells observed following 48 h of Dorsomorphin treatment, by only adding the inhibitor after this period. We treated embryos with 1.0 μM Dorsomorphin from E3.5 to E4.5 and analysed lineage-specific gene expression compared with controls ( Fig. 5g ). This 24 h treatment resulted in a similar decrease in the number of total (by 17%, P <0.05, Student’s t -test) and TE (by 15%, P <0.05, Student’s t -test) cells as in embryos treated for 48 h. PE cell number was reduced by 57% ( P <0.001, Student’s t -test), representing around 60% of the reduction seen with the 48 h treatment. Together, these results suggest that inhibition of the Smad-dependent BMP pathway by Dorsomorphin impairs PE development by two mechanisms. First, by reducing the number of PE precursor cells in the ICM as the early blastocyst forms (E2.5-E3.5), and second, by eliminating Gata6-positive cells by apoptosis in the maturing blastocyst (E3.5-E4.5). (5Z)-7-Oxozeaenol treatment impairs PE cell differentiation The strongest effects on PE development were observed with Dorsomorphin and (5Z)-7-Oxozeaenol, however, our results suggested that these inhibitors might be acting in different ways to reduce PE cell number. To further investigate this hypothesis, we analysed the expression of Gata6 and Nanog in E4.5 embryos treated with 500 nM (5Z)-7-Oxozeaenol from E2.5, compared with controls ( Fig. 6a–c ). Control embryos at this stage had well-sorted PE and EPI cells, with only 5% of ICM cells co-expressing both Gata6 and Nanog. In contrast, 21% of ICM cells in embryos treated with (5Z)-7-Oxozeaenol expressed both genes ( P <0.01, Student’s t -test; Fig. 6c ). The percentage of ICM cells expressing only Gata6 was reduced compared with controls (36% compared with 51%, P <0.01, Student’s t -test), whereas the percentage of ICM cells expressing only Nanog was unchanged (43% compared with 44%). These results suggest that (5Z)-7-Oxozeaenol does not prevent Gata6-positive PE precursor cell specification, but rather prevents efficient downregulation of Nanog and upregulation of later PE genes such as Sox17. The total number of Nanog-positive cells (including those that are also positive for Gata6) in (5Z)-7-Oxozeaenol-treated embryos at E4.5 is therefore significantly increased compared with control embryos (13.6 cells compared with 9.2 cells, P <0.05, Student’s t -test; Fig. 6d ), as observed earlier. This indicates that inhibition of the Smad-independent BMP pathway by (5Z)-7-Oxozeaenol treatment leads to a reduction in the amount of PE formed, not because of an ICM cell fate switch from PE to EPI, but because of a failure of the PE fate programme. 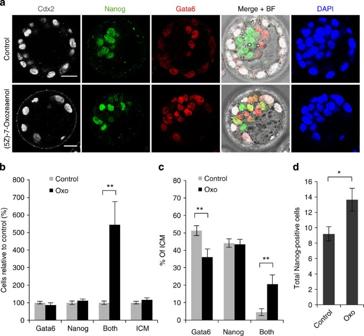Figure 6: (5Z)-7-Oxozeaenol treatment impairs PE cell differentiation. (a–d) Embryos were incubated in the presence of 500 nM (5Z)-7-Oxozeaenol (n=15) for 48 h from E2.5 to E4.5 (controls,n=15). (a) Expression of Cdx2, Gata6 and Nanog at E4.5. Scale bars, 20 μm. (b) Number of cells relative to controls at E4.5. Both=Cells positive for both Gata6 and Nanog. (c) Percentage of ICM at E4.5. (d) Number of Nanog-positive cells at E4.5 (including those also positive for Gata6). *P<0.05, **P<0.01 (Student’st-test). Error bars represent s.e.m. Figure 6: (5Z)-7-Oxozeaenol treatment impairs PE cell differentiation. ( a – d ) Embryos were incubated in the presence of 500 nM (5Z)-7-Oxozeaenol ( n =15) for 48 h from E2.5 to E4.5 (controls, n =15). ( a ) Expression of Cdx2, Gata6 and Nanog at E4.5. Scale bars, 20 μm. ( b ) Number of cells relative to controls at E4.5. Both=Cells positive for both Gata6 and Nanog. ( c ) Percentage of ICM at E4.5. ( d ) Number of Nanog-positive cells at E4.5 (including those also positive for Gata6). * P <0.05, ** P <0.01 (Student’s t -test). Error bars represent s.e.m. Full size image The segregation of cell lineages in the pre-implantation mouse embryo occurs through asymmetric cell divisions that generate outside and inside cells. By analysing the complete transcriptomes of 16-cell stage inside and outside cells, we have identified that components of the BMP signalling pathway are already differentially expressed at this early stage. Most notably, inside cells express the ligands Bmp4 and Bmp7 and outside cells express the receptor Bmpr2 . The differential expression of these genes so early in the development was unexpected as the BMP signalling pathway has not been thought to play a role in pre-implantation development. Indeed, knock-out mice that lack individual components of the BMP pathway have been reported to develop beyond implantation [10] , [11] , [17] , [18] . Differential expression of BMP ligands and receptors in different pre-implantation cell lineages has, however, been observed before, with Bmp4 and Bmp7 found in the ICM and Bmpr2 in the TE at the blastocyst stage [2] , [3] , [32] . Our data therefore show the same pattern of differential expression in the first distinct precursors of these lineages. Gene expression alone does not mean that BMP signalling is active at these stages, however, we show here that nuclear pSmad1, which indicates activity of the Smad-dependent BMP pathway, is present already at the early blastocyst stage ( Fig. 1 ), in agreement with a previous report [27] . To determine whether active BMP signalling is important for pre-implantation development, we used dominant negative forms of Smad4 and Bmpr2. Microinjection of dnSmad4 or dnBmpr2 into one blastomere at the late two-cell stage, thereby inhibiting BMP signalling in half of the embryo from the four-cell stage, resulted in a significant reduction in the number of TE and PE cells in the injected clone at E4.5, but did not affect the embryonic EPI ( Fig. 2 ), suggesting that BMP signalling is important for the development of these two extra-embryonic lineages. Smad4 and Bmpr2 knock-out embryos are able to develop past implantation; however, they exhibit abnormalities in extra-embryonic tissues and fail to gastrulate [10] , [11] , [17] , [18] . To confirm that BMP signalling is important for the pre-implantation development of the TE and PE lineages, we next cultured embryos in the presence of three different BMP inhibitors as these lineages are first set apart, from the eight-cell stage onwards ( Fig. 3 ). Treatment with all of the inhibitors caused a dose-dependent decrease in the number of PE cells, with the Bmpr1 inhibitor Dorsomorphin having the most severe phenotype, causing a reduction in PE cells by 91% at 1.0 μM concentration. All three inhibitors also impaired development of the TE, although to a lesser extent than dominant negative inhibition of Smad4 or Bmpr2. Because the dominant negative mRNAs were injected into the embryos a day earlier than the start of the inhibitor treatments, we hypothesized that their greater effect on the TE may be due to an early effect before the eight-cell stage. Incubation of embryos with Dorsomorphin from the late two-cell stage confirmed that this was indeed the case as TE cell number was reduced by 54% relative to controls, compared with only 9% when the inhibitor was added at E2.5 ( Fig. 3 ). The effect of Dorsomorphin treatment on the PE lineage was not influenced by the longer incubation, with both treatment times resulting in a reduction of PE cells of around 90%. It is therefore likely that the reduction of PE cells represents a slightly later phenotype of BMP inhibition than that of TE cells, probably because the PE lineage is specified later in development. The observed effects on these more differentiated lineages could potentially result from an impaired differentiation process. BMP4 has been shown to be able to induce the differentiation of ES cells into TE and PE in vitro [16] , [34] . Although the differentiation of ES cells is not a direct model for the differentiation of pluripotent blastomeres, it is possible that similar mechanisms could be involved. The Bmp4-induced Smad pathway activates expression of the TE transcriptional programme in ES cells through the interaction of pSmad1 with an evolutionary conserved enhancer region in intron 1 of Cdx2 (ref. 16 ). The expression of Bmpr2 in outside cells at the 16-cell stage could relate to a role of BMP signalling in the development of the extra-embryonic lineages because outside cells at the 16-cell stage are progenitors of both the TE and PE. Indeed, the inside daughters of 16-cell stage outside cells are biased towards a PE fate [6] , [35] . An important question is why these pre-implantation phenotypes have not been observed when studying knock-out mice that lack BMP signalling pathway components. Many inhibitor-treated embryos, despite severely compromised PE and TE lineages, were able to hatch and therefore would most likely be able to implant. An early effect of BMP signalling inhibition on blastocyst development could therefore have been missed in knock-out embryos if the cells in each lineage were not counted before implantation. In addition, it is also possible that an early phenotype may have been masked by the influence of maternal factors in the oviduct and uterus. To investigate how the number of extra-embryonic cells becomes decreased following BMP inhibitor treatment, we examined the embryos for apoptotic cells ( Fig. 4 ). We found evidence of increased levels of apoptosis in embryos treated with Noggin and Dorsomorphin, indicating that programmed cell death is responsible, at least in part, for the decrease in TE and PE cells. Interestingly, treatment with (5Z)-7-Oxozeaenol, which inhibits an alternative Smad-independent downstream pathway, was not associated with an increased incidence of cell death. Moreover, treatment with (5Z)-7-Oxozeaenol also resulted in an increase in EPI cells, whereas the other two inhibitors did not, and it was the only inhibitor not to reduce total cell number in the blastocyst suggesting that it impairs pre-implantation development by an alternative mechanism to Noggin and Dorsomorphin. To determine whether the BMP signals important for the development of the extra-embryonic lineages are generated by inside or outside cells, we knocked-down expression of Bmp4 and Bmp7 ( Fig. 4 ) as these ligands are expressed exclusively by inside cells at the 16-cell stage and by ICM cells in the blastocyst [2] , [3] , [32] . Depletion of these ligands alone resulted in a decrease in the number of TE and PE cells, consistent with the inhibition of BMP signalling. This suggests that BMP signals produced by the pluripotent inside cells are critical for regulating the development of the extra-embryonic TE and PE. Outside cells also express Bmp ligands, so an involvement of autocrine BMP signalling in their development cannot be excluded; however, the dramatic reduction of extra-embryonic cells in Bmp4+7 siRNA embryos suggests that these inside-produced signalling molecules are the predominant ligands involved. The effect of BMP inhibition on the PE lineage is particularly interesting as the earliest phenotype reported in Smad4 knock-out mice is abnormal visceral endoderm, a tissue derived from the pre-implantation PE [17] . These embryos are reduced in size, have secondary defects in gastrulation and die by E7.5. In embryos treated with Dorsomorphin, Sox17-positive PE cells were almost completely absent. To determine whether this is the result of a failure of PE cell specification, a defect in PE differentiation or specific elimination of PE precursor cells, we analysed the expression of Gata6 after Dorsomorphin treatment at both the early (E3.5) and late (E4.5) blastocyst stages ( Fig. 5 ). Gata6 is the earliest marker of PE precursor cells [36] , [37] and therefore the presence of cells in the E4.5 ICM that are positive for Gata6 but negative for Sox17 would imply a fault in the PE transcriptional programme. We found that Gata6-positive cells were reduced by 78% in Dorsomorphin-treated embryos at E4.5, indicating a lack of PE cells rather than an effect on PE cell differentiation. At E3.5, the number of Gata6-positive cells was significantly less than in controls, although this could possibly be due to a slight developmental delay in these embryos. These results, along with the presence of dead and dying cells on the surface of the ICM at E4.5 ( Fig. 5 ), suggest that Dorsomorphin treatment reduces the number of PE cells in the pre-implantation embryo primarily through apoptosis of PE precursors during blastocyst maturation from E3.5 to E4.5, but also reduces the number of PE precursors specified in the early ICM. The greater effect of Dorsomorphin treatment on PE cell number compared with injection of dnSmad4 or dnBmpr2 most likely relates to degradation of the injected mRNAs over time so that they had a lesser effect in later pre-implantation stages. It is also relevant that the dominant negatives were expressed only in half of the embryo and therefore a potential influence of the non-injected half of the embryo on the injected clone of cells cannot be excluded. Embryos treated with (5Z)-7-Oxozeaenol had an increased number of Nanog-positive cells at E4.5 and did not have an increased incidence of apoptosis, suggesting that (5Z)-7-Oxozeaenol impairs development of the PE by a different mechanism to Dorsomorphin. By analysing Gata6 and Nanog expression in (5Z)-7-Oxozeaenol-treated embryos, we discovered that in these embryos PE precursor cells fail to downregulate Nanog and activate the later PE fate transcriptional programme ( Fig. 6 ), indicating that BMP signalling is important for multiple aspects of PE cell development that are possibly mediated by different downstream pathways ( Fig. 7 ). In conclusion, through the use of chemical inhibitors, Bmp-specific siRNAs and the expression of dominant negative components of the BMP pathway, we have uncovered an unexpected role of BMP signalling in the pre-implantation development of extra-embryonic cell lineages. 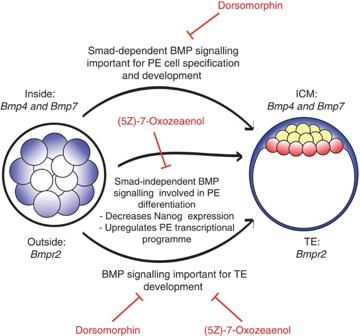Figure 7: Roles of BMP signalling in pre-implantation development. BMP signalling is important for the development of both extra-embryonic cell lineages, the TE and PE. Inhibitors of both the Smad-dependent (Dorsomorphin) and Smad-independent ((5Z)-7-Oxozeaenol) BMP pathways impair development of the TE but have different effects on the PE. Blocking the Smad-dependent pathway results in the elimination of PE precursor cells, while blocking the Smad-independent pathway compromises the differentiation of PE cells. Figure 7: Roles of BMP signalling in pre-implantation development. BMP signalling is important for the development of both extra-embryonic cell lineages, the TE and PE. Inhibitors of both the Smad-dependent (Dorsomorphin) and Smad-independent ((5Z)-7-Oxozeaenol) BMP pathways impair development of the TE but have different effects on the PE. Blocking the Smad-dependent pathway results in the elimination of PE precursor cells, while blocking the Smad-independent pathway compromises the differentiation of PE cells. Full size image Embryo culture and inhibitor treatments Animals were maintained in the Gurdon Institute Animal Facility and all experiments were conducted in compliance with Home Office regulations. Mouse embryos were collected from 4- to 6-week-old F1 (C57Bl6 × CBA) females superovulated with 7.5 IU of pregnant mares’ serum gonadotropin (Intervet) and 7.5 IU human chorionic gonadotropin (Intervet) 48 h later, and mated with F1 males. Embryos were isolated in M2 medium containing 4 mg ml −1 of BSA and cultured in KSOM medium (Millipore) as described previously [21] . The following inhibitors were used: Mouse recombinant Noggin (ProSpec), Dorsomorphin (Tocris Bioscience) (5Z)-7-Oxozeaenol (Tocris Bioscience) and actinomcyin D (Sigma). All inhibitors were dissolved in dimethylsulphoxide. Dimethylsulphoxide diluted in KSOM to an equivalent volume to the highest concentration of inhibitor was used for controls. Human recombinant BMP4 (Sigma) was added to the medium where indicated at a concentration of 100 ng ml −1 . Isolation of cells for mRNA-sequencing Embryos were collected into M2 medium at the four-cell stage and their progression to the eight-cell stage was monitored. Embryos were grouped based on the time they entered the 8-cell stage and embryos in the same group were observed to have undertaken 8- to 16-cell divisions before being incubated in M2 with a fluorescently labelled 0.2 μm microsphere suspension (Polysciences, Inc.) diluted to 1:50 for 30 s. This brief incubation ensures that only outside cells are sufficiently bound by the beads. Embryos were subsequently disaggregated in divalent cations-free M2 medium with gentle pipetting. Outside (strongly fluorescent) and inside (non-fluorescent) cells were isolated, released into cell lysis buffer (PicoPure RNA isolation kit, Arcturus) and frozen on dry ice. SOLiD sequencing and data pre-processing Purified RNA was subjected to the mRNA-seq protocol as described in detail elsewhere [19] . Briefly, oligo(dT)-primed cDNA was generated and amplified representing approximately 1 kb coverage at the 3′ end of all polyadenylated transcripts. SOLiD 4 machine (Applied Biosystems) was used to produce 50-base colour-space reads. Greater than 90 million reads for each of the two libraries was generated and greater than 35 million of each uniquely mapped to the genome. Reads were mapped to the mouse genome (v. NCBI137/mm9) using Bioscope software (Applied Biosystems). Normalization was carried out for sequencing depth (the total number of uniquely aligned reads). qRT–PCR of inside and outside cells For analysis of gene expression at the 16-cell stage, qRT–PCR was performed on the Fluidigm platform following RNA amplification as described earlier [2] using RNA isolated from three to four cells of the same kind (inside or outside from 16-cell stage embryos, isolated as above). Expression of actin B mRNA was used for normalization. Relative expression in inside (9 replicates) and outside (14 replicates) cells was calculated using ΔΔCt method. Immunofluorescence Immunofluorescence was carried out as described previously [38] . Briefly, embryos were fixed in 4% paraformaldehyde, washed in PBS-T (PBS containing 0.1% Tween) and permeabilized with 0.5% Triton X-100 for 20 min. Embryos were incubated with primary antibodies in 3% BSA (Sigma) in PBS-T overnight at 4 °C. The embryos were then washed twice in PBS-T and incubated with secondary antibodies (Invitrogen, AlexFluor; 1:400 in 3% BSA) for 2 h before final washes in PBS-T and M2, and imaging in drops of M2 on glass-bottomed dishes. Primary antibodies used were goat anti-Sox17 (R&D Systems), mouse anti-Cdx2 (Biogenex), rabbit anti-Nanog (2B Scientific), goat anti-Gata4 (Santa Cruz), goat anti-Gata6 (R&D Systems), mouse anti-Oct4 (Santa Cruz), rabbit anti-pSmad1 (Cell Signaling) and rabbit anti-cleaved Caspase 3 (R&D Systems). 4',6-Diamidino-2-phenylindole was used as the nuclear counterstain in all experiments and all primary antibodies were used at a dilution of 1:200. Multichannel images were acquired for multiple sections using a Leica SP5. Image processing and cell counting were performed with Fiji software ( http://fiji.sc ). Microinjection of pre-implantation embryos A dominant negative form of Smad4 ( dnSmad4 ) [39] was cloned downstream of the TagRFP protein in pRN3P as described previously [40] . A dominant negative form of Bmpr2 ( dnBmpr2 ) [41] was cloned upstream of the Ruby protein. To express the dominant negative proteins, one blastomere of two-cell stage embryos was injected with dnSmad4 or dnBmpr2 mRNA (500 ng μl −1 ) and Gap43-RFP mRNA (400 ng μl −1 ) as a marker of injection. Control embryos were injected with Gap43-RFP mRNA alone. Embryos were fixed at E4.5 and the lineage contributions of Gap43-RFP-expressing cells assessed by immunofluorescence. To deplete expression of Bmp4 and Bmp7 in the embryo, two-cell stage embryos were injected into both blastomeres with a combination of four siRNAs (two each targeting Bmp4 and Bmp7 ) at a total concentration of 16 μM. Controls were injected with 16 μM AllStars Negative Control siRNA (Qiagen) and all embryos were co-injected with 100 ng μl −1 of Gap43-GFP mRNA as an injection control. The embryos were fixed at E4.5 and the number of cells in each lineage assessed by immunofluorescence. The siRNA sequences are as follows: Bmp4 siRNA 1: 5′- GCGGTCCAGGAAGAAGAATAA-3′ , Bmp4 siRNA 2: 5′- AGGAGTTTCCATCACGAAGAA-3′ , Bmp7 siRNA 1: 5′- CGGGAGATCCTGTCCATCTTA-3′ , Bmp7 siRNA 2: 5′- CAGCTCTAATGTCATCCTGAA-3′ . qRT–PCR for analysis of siRNA efficiency For confirmation of knockdown, embryos were collected 48 h after siRNA injections (E3.5). Total RNA was extracted using the Arcturus PicoPure RNA Isolation Kit and qRT–PCR was performed using the Power SYBR Green RNA-to-CT 1-Step Kit (Life Technologies) and a StepOne Plus Real-time PCR machine (Applied Biosystems). Relative levels of transcript expression were assessed by the ΔΔCt method, with Gapdh as an endogenous control. The following primers were used: Bmp4 5′- TCTAGAGGTCCCCAGAAGCA -3′, 5′- AGGAATCATGGTGTCTTGACAGA -3′ and Gapdh 5′- AGAGACGGCCGCATCTTC -3′, 5′- CCCAATACGGCCAAATCCGT -3′. Time-lapse imaging Eight-cell stage embryos from F1 × GFP-GPI [42] matings were cultured in KSOM with or without Dorsomorphin for 48 h. Green fluorescence and transmitted light multi-section images were acquired every 20 min using a spinning disk confocal microscopy system and analysed using SlideBook software (3i Intelligent Imaging Innovations). How to cite this article : Graham, S. J. L. et al . BMP signalling regulates the pre-implantation development of extra-embryonic cell lineages in the mouse embryo. Nat. Commun. 5:5667 doi: 10.1038/ncomms6667 (2014). Accession codes: NCBI BioSample accession numbers are SAMN03098868 (outside cells) and SAMN03098869 (inside cells). Sequencing data have been deposited in the NCBI short read archive under BioProject ID PRJNA263313 .